A zero-strain layered metal oxide as the negative electrode for long-life sodium-ion batteries Room-temperature sodium-ion batteries have shown great promise in large-scale energy storage applications for renewable energy and smart grid because of the abundant sodium resources and low cost. Although many interesting positive electrode materials with acceptable performance have been proposed, suitable negative electrode materials have not been identified and their development is quite challenging. Here we introduce a layered material, P2-Na 0.66 [Li 0.22 Ti 0.78 ]O 2 , as the negative electrode, which exhibits only ~0.77% volume change during sodium insertion/extraction. The zero-strain characteristics ensure a potentially long cycle life. The electrode material also exhibits an average storage voltage of 0.75 V, a practical usable capacity of ca. 100 mAh g −1 , and an apparent Na + diffusion coefficient of 1 × 10 −10 cm −2 s −1 as well as the best cyclability for a negative electrode material in a half-cell reported to date. This contribution demonstrates that P2-Na 0.66 [Li 0.22 Ti 0.78 ]O 2 is a promising negative electrode material for the development of rechargeable long-life sodium-ion batteries. With the tremendous development of renewable energies such as solar and wind power, the smooth integration of these energies into the grid, thus improving the grid reliability and utilization, critically needs large-scale energy storage systems with long-life, high efficiency, high safety and low cost [1] , [2] . Among the various energy storage technologies, electrochemical approach represents one of the most promising means to store electricity in large-scale because of the flexibility, high energy conversion efficiency and simple maintenance [2] , [3] , [4] . Because of the highest energy density among practical rechargeable batteries, lithium-ion batteries have been widely used in portable electronic devices and would undoubtedly be the best choice for (hybrid) electric vehicles [5] , [6] . However, the high cost and limited resources of lithium have caused some concerns of using lithium-ion batteries in the large-scale energy storage systems [7] , [8] , [9] , [10] , [11] , [12] , [13] , [14] , [15] . In this background, room-temperature sodium-ion batteries with lower energy density compared with lithium-ion batteries have been reconsidered particularly for such large-scale applications [16] , [17] , [18] , [19] , [20] , [21] , [22] , [23] , [24] , where cycle life and cost are the more essential factors than energy density, in both academic and industrial communities, owing to the abundant sodium resources and potentially low cost as well as the similar ‘rocking-chair’ sodium storage mechanism to that of lithium. Searching for suitable electrode materials to satisfy the long-term stability requirement is an important step to realize the large-scale energy storage. The electrode materials with small volume change during guest ion insertion and extraction, for example, zero-strain characteristics, have attracted great attention because of the potentially excellent long cycling performance. A typical example of zero-strain [25] , [26] negative electrode material is the well-known spinel Li 4 Ti 5 O 12 via a two-phase storage mechanism (Li 4 Ti 5 O 12 and Li 7 Ti 5 O 12 , the volume change between them is ~0.2%), which has been demonstrated for thousands of cycles in lithium-ion batteries [27] , indeed showing the advantage of using zero-strain material for long-term stable cycling. So far to the best of our knowledge, no zero-strain negative electrode material is available for sodium-ion batteries although a few types of negative electrode materials have been reported to be active in sodium-ion batteries [9] , [10] , [11] , [12] , [28] , [29] , [30] , [31] , [32] , [33] , [34] , [35] , [36] , [37] , [38] , [39] , [40] , [41] . Among the available negative electrode materials, hard carbon shows the best overall storage performance in terms of high storage capacity and good cycling. However, most of the capacity is located at the voltage below 0.1 V, which is too close to the sodium plating voltage, causing potential safety concerns, especially at fast charging rates or overcharging. Several oxides such as Na 2 Ti 3 O 7 and alloys (Sn or Sb) have shown high storage capacity [30] , [33] , [34] , [35] , but would not be suitable for long-life batteries owing to the large volume change during sodium insertion and extraction [39] , which is undesirable to the structural stability. Recently, several layered Na x MO 2 (M: 3d transition metals, TMs) compounds have been proposed as positive electrode materials for sodium-ion batteries [42] , [43] , [44] , [45] , [46] , [47] , [48] , [49] , [50] , [51] , [52] . It has also been demonstrated that P2-type materials show better storage performance than that of O3-type materials (Note that the notations of P2 and O3 were defined by Delmas et al . [53] , they refer to different ways of the stacking of the oxygen layer, for example, ABBA for P2, ABCABC for O3 and so on) [46] . In the case of P2-type materials, the value of ‘ x ’ in Na x MO 2 is less than 1 and typically 2/3, leaving many vacancies in the alkali layer. These vacancies could be filled again by sodium insertion, and thus P2-type materials could be used as negative electrodes if the operation potential of TM redox couple is suitable. Among 3d TMs, some Ti oxides show lower redox potential compared with Mn, Fe, Co and Ni oxides [25] , [26] , [27] , [30] , [31] , [32] ; however, TiO 6 octahedral is not stable in air in layered Na 2/3 TiO 2 because of the Ti 3+ environment (note that the electrochemical behaviour of O3-NaTiO 2 which is not stable in air has been reported in 1980s (ref. 54 ). Only 0.3 Na (78 mAh g −1 ) can be reversibly extracted and inserted in this O3-type material.). Introducing ions with lower valence state into Ti sites may increase the valence state of Ti 3+ to Ti 4+ without destroying the layered structure, and may result in the stability of the new compound. Considering the similar ionic radius of Li + and Ti 4+ , we choose Li as a candidate doping element for Na 2/3 TiO 2 . Following this idea, we explored the sodium storage performance of Na 0.66 [Li 0.22 Ti 0.78 ]O 2 in which Li and Ti occupy the TM layer, and found the sodium ionic conductivity to be 0.035 S cm −1 at 300 ° C (ref. 55 ). It is expected that 0.34 Na per formula unit can be inserted into this host. Here we report a zero-strain negative electrode material for sodium-ion batteries, the P2-type layered Na 0.66 [Li 0.22 Ti 0.78 ]O 2 , which exhibits an average storage voltage of 0.75 V and a reversible capacity of 116 mAh g −1 . The most desirable property is that the volume change during sodium insertion and extraction is ~0.77%, showing the zero-strain characteristics, thereby ensuring potentially long cycle life as demonstrated by over 1,200 repeated cycles with capacity retention of 75%. Structure of Na 0.66 [Li 0.22 Ti 0.78 ]O 2 This compound was prepared by a simple solid-state reaction using precursors of Na 2 CO 3 , Li 2 CO 3 and TiO 2 . Fig. 1a shows the synchrotron X-ray diffraction (XRD) pattern and the Rietveld refinement of the resulting material. All of the diffraction peaks are in good agreement with the JCPDS No. 52-0689 and is isostructural with a typical P2-type Na 2/3 CoO 2 (ref. 44 ), indicative of a pure P2 phase material. The Rietveld refinement within a space group of hexagonal P6 3 /mmc gives the lattice parameters of a = b =2.9643(1) Å, c =11.1351(4) Å and V =84.73 Å 3 , which are in good agreement with the ab initio simulation (detailed information is shown in Supplementary Table S1 ). According to the refinement, a schematic structure of the Na 0.66 [Li 0.22 Ti 0.78 ]O 2 is presented in Fig. 1b . Different from O3-type material, the repulsive Coulomb interaction of the AA-type oxygen stacking gives rise to a larger interlayer of 5.5636(5) Å, which was deduced from (002) peak. In this structure, the larger sodium ions occupy the trigonal prismatic sites in one layer, whereas smaller Li and Ti ions co-occupy the neighbouring layer. In addition, some of Na ions (0.425) occupy the 2d site sharing the edges with the TiO 6 octahedra, whereas others (0.211) occupy the 2b site sharing two faces with the TiO 6 octahedra ( Supplementary Table S1 ). This situation is similar to other P2 materials [44] , [48] , [49] , [56] . The morphology of the sample was investigated with scanning electron microscopy. As shown in the inset of Fig. 1a , the distribution of particle size of the as-prepared sample is in the range of 10–15 μm. 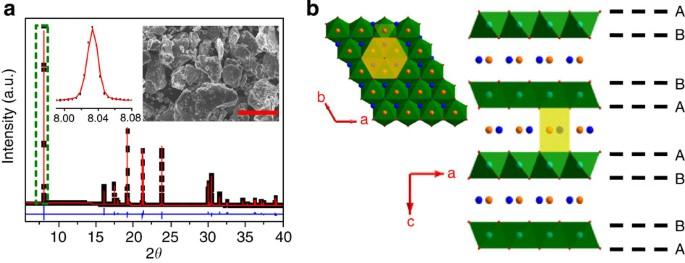Figure 1: Structure of P2-Na0.66[Li0.22Ti0.78]O2. (a) Synchrotron XRD pattern and Rietveld refinement of the as-prepared Na0.66[Li0.22Ti0.78]O2sample. The red (black) line represents the experimental (calculated) data. The residual discrepancy is shown in blue. The refinement is preformed in the P63/mmc space group. The inset is the typical scanning electron micrograph of the as-prepared sample (scale bar is 10 μm). (b) Schematic illustration of the hexagonal Na0.66[Li0.22Ti0.78]O2projected ina-cplane (left top is projected ina-bplane). Symbols A and B refer to the different oxygen layers. The green layer represents the Ti(Li)O2layer and orange (2b site) or blue (2d site) bullets refer to Na ions that occupy the trigonal prismatic sites between two Ti(Li)O2layers. Figure 1: Structure of P2-Na 0.66 [Li 0.22 Ti 0.78 ]O 2 . ( a ) Synchrotron XRD pattern and Rietveld refinement of the as-prepared Na 0.66 [Li 0.22 Ti 0.78 ]O 2 sample. The red (black) line represents the experimental (calculated) data. The residual discrepancy is shown in blue. The refinement is preformed in the P6 3 /mmc space group. The inset is the typical scanning electron micrograph of the as-prepared sample (scale bar is 10 μm). ( b ) Schematic illustration of the hexagonal Na 0.66 [Li 0.22 Ti 0.78 ]O 2 projected in a - c plane (left top is projected in a - b plane). Symbols A and B refer to the different oxygen layers. The green layer represents the Ti(Li)O 2 layer and orange (2b site) or blue (2d site) bullets refer to Na ions that occupy the trigonal prismatic sites between two Ti(Li)O 2 layers. Full size image Sodium storage performance The sodium storage performance of P2-Na 0.66 [Li 0.22 Ti 0.78 ]O 2 in sodium half cells is shown in Fig. 2a . In the first discharge curve, it can be seen that the voltage drops quickly to 1.2 V and then decreases monotonically from 1.2 to 0.4 V, indicating the sodium insertion through a solid-solution reaction [44] . (note that the reason of choosing the cut-off voltage of 0.4 V is that it delivers the best cyclic performance as shown in Supplementary Fig. S1 ). This is further supported by the synchrotron in situ XRD results as discussed later. This behaviour is different from other P2-type electrodes, where multiple plateaus were usually observed during sodium extraction/insertion which is related to a series of phase transitions (sodium/vacancy ordering or charge ordering) [9] , [10] , [11] , [12] , [44] , [48] . The random distribution of Li in the TM layer, which is deduced from the high resolution XRD pattern that does not exhibit any superstructure peaks [49] , could be responsible for such sodium storage mechanism in the P2-Na 0.66 [Li 0.22 Ti 0.78 ]O 2 . The other feature of interest is that the average sodium storage voltage is ca. 0.75 V, higher than that of layered Na 2 Ti 3 O 7 (0.3 V) [30] which is close to the sodium plating voltage, making it much safer. 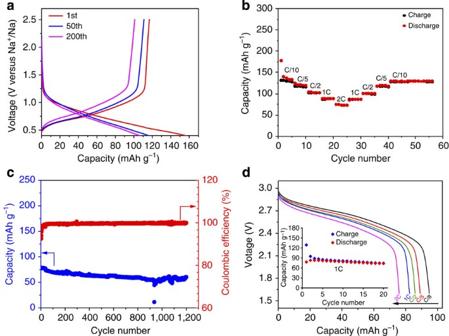Figure 2: Sodium storage performance of P2-Na0.66[Li0.22Ti0.78]O2electrodes. (a) The 1st, 50th and 200th discharge/charge curves at a current rate of C/10 (10.6 mA g−1) in the voltage range of 0.4 and 2.5 V versus Na+/Na. (b) Rate capability. The capacity versus cycle number at various current rates. (c) Long-term cycling performance. The capacity and Coulombic efficiency versus cycle number at a current rate of 2C. (d) Discharge profiles of Na0.66[Li0.22Ti0.78]O2//Na3V2(PO4)3/C sodium-ion full cell at various rates (inset is the cyclic performance of the full cell at 1C rate). The average potential of sodium insertion into P2-Na x [Li 0.22 Ti 0.78 ]O 2 (0.66≤ x ≤1) can be estimated as: Figure 2: Sodium storage performance of P2-Na 0.66 [Li 0.22 Ti 0.78 ]O 2 electrodes. ( a ) The 1st, 50th and 200th discharge/charge curves at a current rate of C/10 (10.6 mA g −1 ) in the voltage range of 0.4 and 2.5 V versus Na + /Na. ( b ) Rate capability. The capacity versus cycle number at various current rates. ( c ) Long-term cycling performance. The capacity and Coulombic efficiency versus cycle number at a current rate of 2C. ( d ) Discharge profiles of Na 0.66 [Li 0.22 Ti 0.78 ]O 2 //Na 3 V 2 (PO 4 ) 3 /C sodium-ion full cell at various rates (inset is the cyclic performance of the full cell at 1C rate). Full size image in which E is the theoretical total energy per f.u. obtained from density functional theory (DFT) calculations. Entropy and temperature effects are not considered. The calculated average potential is 0.47 V, which is slightly lower than the experimental value. The difference may come from the absence of kinetic effects in the calculations, where the potential we obtained is thermodynamic equilibrium voltage. The reversible capacity is 116 mAh g −1 , corresponding to 0.38 Na insertion per formula unit. This value is slightly higher than the available vacancy (0.34) in the Na 0.66 [Li 0.22 Ti 0.78 ]O 2 . Note that the inductively coupled plasma-optical emission spectrometer result shows the real composition of the resulting material is Na 0.63 [Li 0.22 Ti 0.78 ]O 1.98 , leaving some sodium and oxygen vacancies. In this case, it will allow 0.37 Na insertion into the host, corresponding to a capacity of 116 mAh g −1 , which is close to what we obtained. An irreversible capacity loss was observed in the first cycle, which could be ascribed to the formation of solid electrolyte interphase layer (SEI) when discharged to a lower voltage ( Supplementary Fig. S2 ). This is a common phenomenon in the lithium-ion batteries for a low voltage negative electrode. The electrode can also be cycled well at 60 ° C ( Supplementary Fig. S3 ). The rate capability of the Na 0.66 [Li 0.22 Ti 0.78 ]O 2 electrode was also evaluated in a sodium cell. It can be seen from Fig. 2b that the reversible capacities are 116, 106, 90, 77 and 62 mAh g −1 at constant current rates of C/10, C/5, C/2, 1C and 2C, respectively. The capacity retention at 2C is 53.4% of the initial capacity. It should be noted that these values were obtained from the sample with pretty large particle size (10–15 μm) and without any special efforts such as carbon-coating and nanosizing. We believe the rate capability could be further optimized. The most appealing property of this material is the excellent long-term cyclic stability. As shown in Fig. 2c and Supplementary Fig. S4 , the Na 0.66 [Li 0.22 Ti 0.78 ]O 2 electrode exhibits over 1,200 cycles with capacity retention of 75% at a current rate of 2C (a very small capacity decay of 0.02% per cycle). The Coulombic efficiency after initial cycles can reach nearly 100%. (note that the low Coulombic efficiency at initial cycles is probably related to the electrolyte degradation and/or unstable metallic sodium electrode [14] , [21] , [57] ). Both parameters are crucial for a practical application. As far as we know, P2-Na 0.66 [Li 0.22 Ti 0.78 ]O 2 exhibits the best cycling performance demonstrated so far among all reported negative electrode materials for sodium-ion batteries [28] , [29] , [30] , [31] , [32] , [33] , [34] , [35] , [36] . A sodium-ion full cell was also demonstrated using P2-Na 0.66 [Li 0.22 Ti 0.78 ]O 2 as negative electrode and Na 3 V 2 (PO 4 ) 3 /C as positive electrode. In order to obtain a practical usable capacity for full cell, the electrode was also cycled in a narrow voltage range of 0.4–1.4 V ( Supplementary Fig. S5 ). It can be seen that a reversible capacity of ca. 100 mAh g −1 can be achieved. Preliminary results show that the full cell gives rise to an average operating voltage at ~2.5 V and appropriate rate and cycling performance ( Fig. 2d ). The performance can be further enhanced by optimization of both electrodes and their weight ratio. To understand the structure evolution during sodium insertion and extraction, we performed the synchrotron electrochemical in situ XRD experiment and the results are plotted in Fig. 3 (also see Supplementary Fig. S6 ). No new peaks beyond P2 structure were observed at the beginning of sodium insertion, but only some slightly shift to higher two theta angles and others to lower angle upon sodium insertion. In particular, the shift of the (002) peak is very small. It can be observed that a solid-solution reaction apparently occurs at the initial discharge until 0.55 V, evidenced by a continuous peak shift and lattice constant variation ( Supplementary Fig. S7 ), with the structure being identified with a single P2 phase. However, along with further sodium insertion, it is interesting to find the shape of (002) peak becomes asymmetry with a broad feature, which is indicative of multiphase or domains. In order to make this point clear, a long-time XRD measurement was carried out on the finally discharged electrode (discharged to 0.4 V, sample was scratched off from the electrode and loaded into capillary) and a high resolution XRD pattern was obtained ( Fig. 4a ). It can be seen that the resulting XRD pattern can be fitted very well with two P2-Na x Li 0.22 Ti 0.78 O 2 phases with very similar cell parameters: ( a = b =2.9932(0) Å, c =10.9538(3) Å) and ( a = b =3.0066(1) Å, c =10.9087(5) Å). The discrepancy between these two phases is mainly caused by the Na occupancy difference within the unit cell (the detailed structure information is presented in Supplementary Table S1 ). One may doubt that this result originated from the experimental technique error because it is well-known that the reduced Ti-based oxides are very easy to get oxidized, either through contact with air or by reacting with organic solvent [54] . In order to avoid the sample "change" during ex situ sample preparation, a newly developed technique based on a combination of chemical sodiation and in situ synchrotron XRD was further performed. The most advantage of this new technique is that during the X-ray measurement the sample in capillary will not be exposure to air. The in situ XRD patterns collected during chemical sodiation are presented in Fig. 5 . The sodiation proceeds very quickly, evidenced by the continuous shift of the (002) peak at the initial chemical sodiation stage (0–45 min). Further Na insertion causes a new phase emerge, reflected by the asymmetry of the (002) peak. The similar phase transition behaviour during chemical sodiation further supports our electrochemical in situ XRD results. After chemical sodiation for 60 h, we collected the XRD pattern with a high resolution as shown in Fig. 4b . Similar as the abovementioned ex situ result (discharged 0.4 V sample), the pattern of the fully sodiated product can also not be refined with a single-phase model. After carefully examining the XRD pattern, a multiphase (same space group: P6 3 /mmc) with gradient lattice variation model [58] was adopted in the Rietveld refinement and a very good refinement result was obtained ( Fig. 4b and Supplementary Table S1 ). The major difference between these similar phases is originated from the sodium occupancy difference at the 2d site, which may be mostly due to the inhomogeneous reaction during chemical sodiation (non equilibrium process) compared with electrochemical reaction. The average Na molar concentration estimated from the refinement is ~0.945, slightly smaller than the ICP result (Na 0.99 [Li 0.22 Ti 0.78 ]O 1.98 ), probably owing to the refinement error or non-crystallized phase that cannot be detected by XRD [59] . On the basis of this, we can conclude that the final discharge or sodiated product actually consists of several P2 phases which have slight different Na contents and occupations (2b,2d). It should be pointed out that the amount of Na occupation at 2b site is decreased along with more and more Na insertion. Upon Na insertion, from an electrostatic point of view, Na will preferentially occupy the 2d site in the interslab because 2d site shares the edges with the TiO 6 octahedra and has less electrostatic repulsion between Na and TiO 6 octahedra [44] , [48] , [49] , [56] . After a large amount of Na occupies the 2d site, a part of Na at the 2b site sharing two faces with the TiO 6 octahedra will be pushed to the 2d site due to the strong electrostatic repulsion between 2b and 2d sites (a scheme has been shown in Supplementary Fig. S8 ). 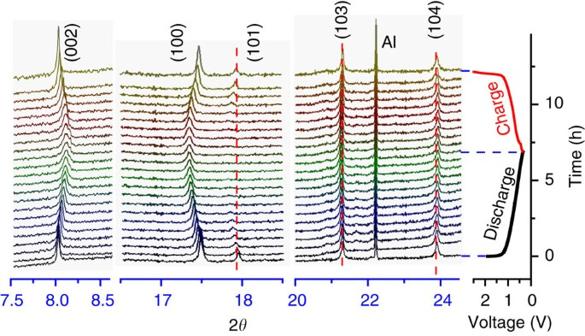Figure 3: Structure evolution of electrochemical sodiation. In situXRD patterns collected during the first discharge/charge of the Na/Na0.66[Li0.22Ti0.78]O2cell under a current rate of C/7 at voltage range between 0.4 and 2.5 V. Figure 3: Structure evolution of electrochemical sodiation. 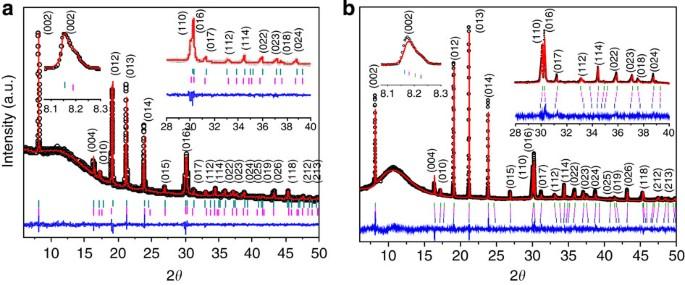Figure 4: Synchrotron XRD patterns and Rietveld refinements. The XRD patterns of (a) the Na0.66[Li0.22Ti0.78]O2electrode discharged to 0.4 V and (b) the Na0.66[Li0.22Ti0.78]O2sample after chemical sodiation for 60 h. They show that the final electrochemically and chemically sodiated samples are actually a mixture of several P2 phases, which may be due to the inhomogeneity of the Na occupancy. The red (black) line represents the experimental (calculated) data. The residual discrepancy is shown in blue. The refinement is preformed in the P63/mmc space group. The Bragg peak positions are shown by the vertical lines. In situ XRD patterns collected during the first discharge/charge of the Na/Na 0.66 [Li 0.22 Ti 0.78 ]O 2 cell under a current rate of C/7 at voltage range between 0.4 and 2.5 V. Full size image Figure 4: Synchrotron XRD patterns and Rietveld refinements. The XRD patterns of ( a ) the Na 0.66 [Li 0.22 Ti 0.78 ]O 2 electrode discharged to 0.4 V and ( b ) the Na 0.66 [Li 0.22 Ti 0.78 ]O 2 sample after chemical sodiation for 60 h. They show that the final electrochemically and chemically sodiated samples are actually a mixture of several P2 phases, which may be due to the inhomogeneity of the Na occupancy. The red (black) line represents the experimental (calculated) data. The residual discrepancy is shown in blue. The refinement is preformed in the P6 3 /mmc space group. The Bragg peak positions are shown by the vertical lines. 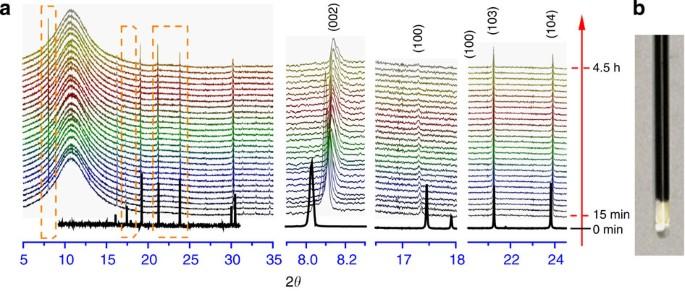Figure 5: Structure evolution of chemical sodiation. (a)In situXRD patterns collected during the chemical sodiation of the Na0.66[Li0.22Ti0.78]O2using sodium-biphenyl-DME reducing agent. (b) A scheme of capillary containing Na reducing agent and the Na0.66[Li0.22Ti0.78]O2sample for thein situXRD experiment. Full size image Figure 5: Structure evolution of chemical sodiation. ( a ) In situ XRD patterns collected during the chemical sodiation of the Na 0.66 [Li 0.22 Ti 0.78 ]O 2 using sodium-biphenyl-DME reducing agent. ( b ) A scheme of capillary containing Na reducing agent and the Na 0.66 [Li 0.22 Ti 0.78 ]O 2 sample for the in situ XRD experiment. Full size image These observations indicate that the sodium insertion in this material is like quasi-solid-solution reaction, which is in good agreement with the shape of discharge curve. After 0.34 Na insertion, it is interesting to note that the P2 phases can still be maintained according to our in situ and ex situ XRD results. On the basis of the refinement results as shown in Table 1 , it can be seen that the c axis is decreased by 2.03%, whereas the a ( b ) axis is expanded by 1.43% after Na insertion, which are in good agreement with DFT calculations. The trend of the change of the lattice parameter during discharge and charge is similar to a typical layered LiCoO 2 . The Coulomb attraction between inserted alkali metal ions and TM layers draws the neighbouring TM layers closer, and the larger ion size of the more reduced TM cations causes the expanded TM-O bond. Nevertheless, the unit-cell volume change before and after sodium insertion is ~0.77%, which is close to zero-strain characteristics. It should be noted that this small volume change is originated from the lattice parameter changes in the opposite directions ( a and b expand, whereas c contracts during Na insertion). This would effectively ensure the structural stability of the electrode during cycling, leading to an excellent long cycle life as demonstrated by over 1,200 cycles. It should be mentioned that this is the first zero-strain negative electrode material for long-life sodium-ion batteries. Table 1 Structural parameters. Full size table No capacity contribution originating from the migration of Li + ions from the TM sites is observed in the experiment. Although the radii of Li + ions is smaller than that of Na + ions, the path connecting two Li + sites is through the TiO 6 octahedra in which the space is too small to accommodate a Li + ion. For this reason, the migration of Li + ions within the [Li 0.22 Ti 0.78 ]O 2 layer will not occur. The Li + ion diffusion from TM layer to the Na layer is also difficult according to the calculated migration energy barrier as shown in Fig. 6 . The energy barrier for Li + ions leaving the TM layer is ~1 eV, whereas the activation energy for Na + ion diffusion within the Na layer is only ~0.4 eV. Accordingly, the estimated diffusion coefficient is ~5.9 × 10 −20 cm −2 s −1 for Li + and ~2.1 × 10 −10 cm −2 s −1 for Na + , indicating that the migration of Li + ions can be ignored compared with that of Na + ions (experimental results are shown in Supplementary Fig. S9 ). Besides the large energy barrier for Li + migration, the occupation of Li at Na site will increase the total energy of the system by ~0.8 eV ( Fig. 6b ), indicating that the migration of Li + ions into Na layer is energetically unfavourable. This can be understood by the different ionic radii of Li + and Na + . This is also supported by the fact that no any Li can be detected from the electrolyte and the sodium electrode according to ICP experiment. The occupation of Li + with smaller radii at the Na site will cause obvious local strain and thus increase the energy of whole system. The detailed migration pathways of Na + ions are analysed using DFT calculations, and the diffusion kinetics comparison between P2- and O3-type structures are shown in Supplementary Fig. S10 and Fig. S11 , which further prove that the trigonal prismatic environment is much more beneficial for the migration of Na + ions. 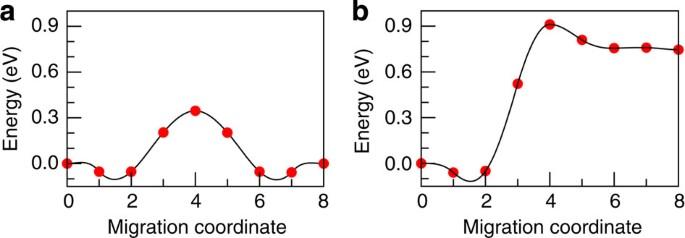Figure 6: DFT calculations. The calculated migration energy barrier of the single vacancy assisted (a) Na+ion diffusion in the Na layer, and (b) Li+ion diffusion from the transition metal layer to the Na layer in P2-Na[Li0.33Ti0.67]O2. Figure 6: DFT calculations. The calculated migration energy barrier of the single vacancy assisted ( a ) Na + ion diffusion in the Na layer, and ( b ) Li + ion diffusion from the transition metal layer to the Na layer in P2-Na[Li 0.33 Ti 0.67 ]O 2 . Full size image In summary, the P2-type layered Na 0.66 [Li 0.22 Ti 0.78 ]O 2 shows a reversible capacity of 116 mAh g −1 at an average storage voltage of 0.75 V which is far from the sodium plating voltage, making the battery potentially safer. The most important appealing feature is the zero-strain characteristics of this material during sodium insertion/extraction, which ensures the long cycle life as demonstrated by over 1,200 cycles with a very small capacity decay of 0.02% per cycle, representing the best cyclic performance so far among all the reported negative electrode materials for sodium-ion batteries. In addition, this P2-type layered material exhibits an unusual quasi-single-phase electrochemical storage behaviour which is in contrast to most of other P2-type materials. We believe that these findings obtained here open a new avenue in the search of even better negative electrode materials and will be helpful in speeding up the development of room-temperature long-life sodium-ion batteries for large-scale energy storage systems. Synthesis The resulting material was prepared by a solid-state reaction using precursors of Li 2 CO 3 (99%), Na 2 CO 3 (99%) and TiO 2 (99.5%, anatase form). A phase-pure compound was obtained when an excess of 2 mol% Li 2 CO 3 and Na 2 CO 3 was used. The starting materials were ground in an agate mortar and pressed into pellets under pressure of 20 MPa. Then the pellets were heated at 1000 ° C for 24 h in an alumina crucible. Characterizations The morphologies of the materials were investigated using a scanning electron microscope (Hitachi S-4800) and a transmission electron microscope (Tecnai G 2 F20 U-TWIN). The XRD patterns were collected in a transition mode at beamline X14A of National Synchrotron Light Source (NSLS, BNL) by a linear position-sensitive silicon detector. The wavelength used was 0.7784 Å. For in situ XRD experiment during electrochemical cycling, CR2032 coin-type cell was used with a glassy carbon window for X-ray penetration; for in situ XRD experiment during chemical sodiation according to our recent work that will be published elsewhere. A total of 0.6 mg Na 0.66 Li 0.22 Ti 0.78 O 2 powder dispersed with cotton was loaded into a glass capillary (0.7 mm in diameter), then, 0.01 ml sodium-biphenyl-DME solution (1 mol Na: 1 mol biphenyl per litre of DME solution) was injected into the capillary. The open end of the capillary was quickly sealed and the capillary was immediately transferred to the synchrotron beamline for in situ experiment. All the operations were carefully performed in the argon-filled glove box. Structures were refined using the Rietveld method as implemented in the TOPAS software package (version 4.1). The background was estimated by chebyshev polynomials. The atomic displacement parameters (ADP or Biso) were fixed to reasonable values (1.0, 0.5, 0.5 and 0.8 Å 2 for sodium, titanium, lithium and oxygen, respectively). Electrochemistry The working electrode was prepared by spreading the slurry of the active materials (60 wt%), acetylene black (30 wt%) and the polyvinylidene fluoride (10 wt%) binder on Cu foil. The working electrodes were dried at 100 ° C under vacuum for 10 h. The electrolyte is 1 M NaClO 4 in EC:DEC (4:6 in volume). The coin-type (CR2032) cells were assembled with pure sodium foil as the counter electrode, and a glass fibre as the separator in an argon-filled glove box. The charge and discharge measurements were carried out on a Land BT2000 battery test system (Wuhan, China) in a voltage range of 0.4–2.5 V under room temperature and 60 ° C. A sodium-ion full cell was constructed using Na 0.66 [Li 0.22 Ti 0.78 ]O 2 as the negative electrode and Na 3 V 2 (PO 4 ) 3 /C as the positive electrode in a CR2032 coin-type cell. The Na 0.66 [Li 0.22 Ti 0.78 ]O 2 electrode was prepared as shown in the above part, and the Na 3 V 2 (PO 4 ) 3 /C electrode was prepared according to our previous report. The weight ratio of the two electrodes (negative/positive) was 1:1.8. The electrolyte solution was 1 M NaPF 6 in EC:DEC (4:6 in volume). The full cells were charged and discharged between the voltage range of 1.6–3.0 V at various C-rates (C/10 current rate corresponds to 10.6 mA g −1 ). Supplementary Fig. S12 shows the first charge/discharge profile of the full cell at a current rate of C/10. DFT calculations The calculations were performed with the Vienna ab initio simulation package. The present data were obtained using the spin-polarized generalized gradient approximation with a parameterized exchange-correlation functional according to Perdew-PBE. The Na(2 p ,3 s ), Li(1 s ,2 s ,2 p ), Ti(3 d ,4 s ) and O(2 s ,2 p ) orbital are treated as valence states. The cutoffs for the wave function and density are 500 eV and 756 eV, respectively. The energy barriers of diffusion pathways were calculated by the nudged elastic band method with the energy and force convergence criterion 10 −5 eV Å −1 and 0.01 eV Å −1 , respectively. How to cite this article: Wang, Y, et al . A zero-strain layered metal oxide as the negative electrode for long-life sodium-ion batteries. Nat. Commun. 4:2365 doi: 10.1038/ncomms3365 (2013).